Depleting the methyltransferase Suv39h1 improves DNA repair and extends lifespan in a progeria mouse model A de novo G608G mutation in LMNA gene leads to Hutchinson–Gilford progeria syndrome. Mice lacking the prelamin A-processing metalloprotease, Zmpste24, recapitulate many of the progeroid features of Hutchinson–Gilford progeria syndrome. Here we show that A-type lamins interact with SUV39H1, and prelamin A/progerin exhibits enhanced binding capacity to SUV39H1, protecting it from proteasomal degradation and, consequently, increasing H3K9me3 levels. Depletion of Suv39h1 reduces H3K9me3 levels, restores DNA repair capacity and delays senescence in progeroid cells. Remarkably, loss of Suv39h1 in Zmpste24 −/− mice delays body weight loss, increases bone mineral density and extends lifespan by ∼ 60%. Thus, increased H3K9me3 levels, possibly mediated by enhanced Suv39h1 stability in the presence of prelamin A/progerin, compromise genome maintenance, which in turn contributes to accelerated senescence in laminopathy-based premature aging. Our study provides an explanation for epigenetic alterations in Hutchinson–Gilford progeria syndrome and a potential strategy for intervention by targeting SUV39H1-mediated heterochromatin remodelling. A de novo G608G mutation in LMNA gene is the predominant cause of Hutchinson–Gilford progeria syndrome (HGPS), an early-onset premature aging disorder [1] , [2] . Lamin A, encoded by the LMNA locus, belongs to type V intermediate filament proteins and is one of the major components of nuclear lamina and nuclear matrix [3] . Lamin A is firstly synthesized as prelamin A with a C-terminal CaaX motif, which dictates a series of processing events including transient isoprenylation, methylation and proteolytic cleavages [4] . ZMPSTE24, a metalloprotease, is required for the second proteolytic cleavage. The G608G mutation activates a cryptic splicing signal, giving rise to a truncated prelamin A termed progerin, which lacks the second proteolytic cleavage site of ZMPSTE24. Loss of Zmpste24 causes accumulation of partially processed prelamin A in mouse embryonic fibroblasts (MEFs), and many of the progeroid features found in HGPS patients are recapitulated in Zmpste24 null mice [5] . Altered nuclear shape is one of the hallmarks of HGPS dermal fibroblasts and cells derived from Zmpste24 –/– embryos [2] , [5] , [6] . Accelerating autophagic degradation of progerin through rapamycin or reducing prelamin A and progerin accumulation on the nuclear envelope by farnesyl transferase inhibitor (FTI) ameliorates senescence in HGPS cells [7] , [8] , [9] , [10] and progeroid features in progeria mouse models [8] , [11] , [12] . We and others have previously shown that γ-H2AX/53BP1 foci accumulate in progeroid fibroblasts and normal senescent human cells, which is now widely used as a cellular marker for HGPS and senescence [6] , [13] , [14] , [15] , [16] , [17] . Upon γ -irradiation, DNA lesions are successfully repaired within 24 h in wild-type cells, whereas a substantial number of the γ-H2AX/53BP1 foci, likely representing unrepaired/irreparable DNA damages, remains in HGPS and Zmpste24 −/− cells [6] . Compromised recruitment of checkpoint response and repair proteins is responsible for defective DNA repair in progeroid cells [6] . However, the underlying molecular mechanism remains largely unknown. Chromatin is highly dynamic and regulated by a variety of binding proteins and complexes to meet the functional requirement in response to various stimuli and stress [18] . Upon DNA damage, the compact chromatin, especially heterochromatin, undergoes global nucleosomal remodelling modulated by ATM-mediated KAP-1 (KRAB-associated protein 1, also known as Trim28 or Tif1β) phosphorylation, resulting in a de-condensed conformation of chromatin accessible to essential DNA repair proteins [19] . Deficiency in ATM leads to accumulation of γ-H2AX/53BP1 foci associated with H3K9me3, a constitutive heterochromatin mark. Knocking down Suv39h1/2, the main methyltransferases responsible for H3K9me3, rescues the defects in heterochromatin remodelling and DNA repair impeded by ATM deficiency [20] . In this study, we investigated whether the defective DNA repair in the presence of progerin/prelamin A is a consequence of abnormal H3K9me3-mediated heterochromatin remodelling. Our data suggest that lamin A interacts with SUV39H1 and protects it from proteasomal degradation. Compared with lamin A, prelamin A/progerin exhibits elevated binding capacity to SUV39H1, leading to increased levels of SUV39H1 and H3K9me3. Depleting Suv39h1 rescues DNA repair and early senescence, ameliorates progeroid features and extends lifespan in Zmpste24 −/− mice. Our data not only implicates a role for lamin A in regulating heterochromatin marked with H3K9me3 but also provides a novel SUV39H1-based therapeutic strategy for HGPS. Sustained DNA damage foci are associated with H3K9me3 To investigate if the defective recruitment of DNA-damage checkpoint response/repair proteins in the presence of progerin/prelamin A is a consequence of abnormal heterochromatin remodelling, we first examined whether the sustained DNA damage foci in HGPS dermal fibroblast cell line HGADFN003 (HG003) after γ-irradiation are associated with H3K9me3. By immunofluorescence staining and confocal microscopy, we found that most of the sustained γ-H2AX/53BP1 foci were associated with regions enriched with H3K9me3 staining at 24 h after γ-irradiation in HG003 cells ( Fig. 1a–c and Supplementary Fig. S1 ), suggesting that condensed heterochromatin marked by H3K9me3 might build up a barrier for the effective DNA repair. To test this hypothesis, we knocked down SUV39 (SUV39H1 and SUV39H2) via short interfering RNA (siRNA) to examine whether this would impact the DNA damage repair. Knocking down SUV39 not only decreased the level of H3K9me3 but also significantly reduced the number of γ-H2AX-containing DNA damage foci in HG003 cells at 24 h after γ-irradiation ( Fig. 1c–e ; 7.67±2.03 γ-H2AX-containing foci in scramble-treated HG003 versus 2.35±1.21 in siSUV39-treated HG003, mean±s.e.m., n >100, P <0.01, two-tailed t -test). The global level of γ-H2AX was also significantly downregulated determined by western blotting ( Fig. 1e ). Knocking down Suv39h1/2 by siRNA had a similar effect in Zmpste24 −/− MEFs on DNA damage foci accumulation at 24 h after γ-irradiation ( Supplementary Fig. S2a–c ); depleting Suv39h1 alone in Zmpste24 −/− MEFs is enough to downregulate the level of H3K9me3 ( Supplementary Fig. S2d ) and reduce the number of DNA damage foci at 24 h after γ-irradiation ( Supplementary Fig. S2e ; 5.4±0.6 53BP1 foci in Zmpste24 −/− Suv39h1 −/− versus 8.1±1.0 in Zmpste24 −/− MEFs, mean±s.e.m., P <0.05, two-tailed t -test). 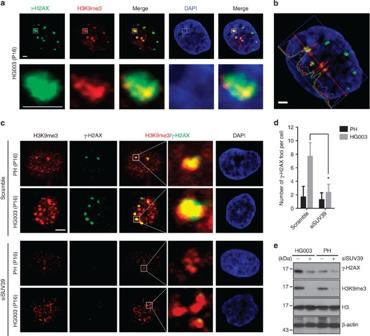Figure 1: Defective heterochromatin repair in HGPS fibroblasts. (a) Representative photos of immunofluorescence staining of H3K9me3 and γ–H2AX in HGPS dermal fibroblast cell line HGADFN003 (HG003) at 24 h after γ-irradiation (5 Gy). Scale bar, 5 μm. (b) Line scans of H3K9me3, γ–H2AX and DAPI signal intensity in the cell shown in (a). Scale bar, 5 μm. (c) Representative photos of immunofluorescence staining of H3K9me3 and γ-H2AX in SUV39 siRNA or scramble-treated HG003 and healthy control cells (PH) at 24 h after γ-irradiation (5 Gy). Scale bar, 10 μm. (d) Quantification of γ-H2AX foci in the experiment ofc. At least 100 cells were counted. Data represent mean±s.e.m., *P<0.05, two-tailedt-test. (e) Representative immunoblots showing levels of H3K9me3 and γ-H2AX in PH and HG003 cells (passage 16) treated with SUV39 siRNA or scramble at 24 h after γ-irradiation (5 Gy). Figure 1: Defective heterochromatin repair in HGPS fibroblasts. ( a ) Representative photos of immunofluorescence staining of H3K9me3 and γ–H2AX in HGPS dermal fibroblast cell line HGADFN003 (HG003) at 24 h after γ-irradiation (5 Gy). Scale bar, 5 μm. ( b ) Line scans of H3K9me3, γ–H2AX and DAPI signal intensity in the cell shown in ( a ). Scale bar, 5 μm. ( c ) Representative photos of immunofluorescence staining of H3K9me3 and γ-H2AX in SUV39 siRNA or scramble-treated HG003 and healthy control cells (PH) at 24 h after γ-irradiation (5 Gy). Scale bar, 10 μm. ( d ) Quantification of γ-H2AX foci in the experiment of c . At least 100 cells were counted. Data represent mean±s.e.m., * P< 0.05, two-tailed t -test. ( e ) Representative immunoblots showing levels of H3K9me3 and γ-H2AX in PH and HG003 cells (passage 16) treated with SUV39 siRNA or scramble at 24 h after γ-irradiation (5 Gy). Full size image Increased levels of Suv39h1 and H3K9me3 in progeroid cells To evaluate whether SUV39H1 directly contributes to the defective DNA repair and delayed recruitment of checkpoint response/repair proteins in progeria, we examined the levels of Suv39h1 protein and mRNA in Zmpste24 –/– MEFs and in cells with ectopic progerin. Suv39h1 protein level was significantly increased in MEFs and tissues isolated from Zmpste24 –/– mice and in HEK293 cells expressing ectopic progerin in comparison with those isolated from littermate wild-type controls and cells expressing ectopic lamin A ( Fig. 2a–d ). In contrast, levels of Suv39h1 mRNA were hardly affected in MEFs and HEK293 cells stably expressing different ectopic lamins analysed by real-time PCR ( Supplementary Fig. S3 ). These suggest that prelamin A and progerin regulate Suv39h1 stability post-translationally. 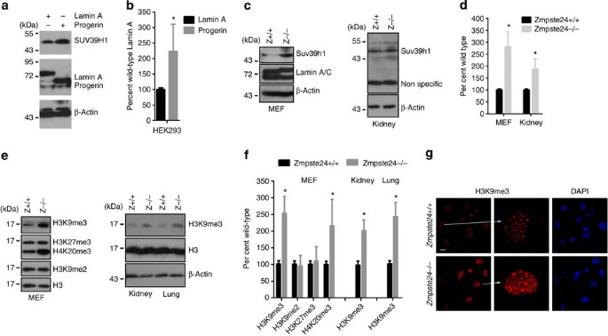Figure 2: Increased levels of Suv39h1 and H3K9me3 in progeroid cells. (a) Representative immunoblots showing the level of SUV39H1 in HEK293 cells expressing ectopic lamin A or progerin. (b) Quantification of experiments ina. Data represent mean±s.e.m.,n=3. *P<0.05, two-tailedt-test. (c) Representative western blotting showing the level of Suv39h1 in wild-type andZmpste24−/−MEFs and in kidney from wild-type andZmpste24−/−mice. (d) Quantification of experiments inc. Data represent mean±s.e.m.,n=3. *P<0.05, two-tailedt-test. (e) Representative immunoblots showing levels of different histone modifications in total cell lysate from wild-type andZmpste24−/−MEFs and indicated wild-type andZmpste24−/−tissues. (f) Quantification of experiments ine. Data represent mean±s.e.m.,n=3. *P<0.05, two-tailedt-test. (g) Representative photos of immunofluorescence staining of H3K9me3 in wild-type andZmpste24−/−MEFs. Scale bar, 20 μm. Figure 2: Increased levels of Suv39h1 and H3K9me3 in progeroid cells. ( a ) Representative immunoblots showing the level of SUV39H1 in HEK293 cells expressing ectopic lamin A or progerin. ( b ) Quantification of experiments in a . Data represent mean±s.e.m., n =3. * P< 0.05, two-tailed t -test. ( c ) Representative western blotting showing the level of Suv39h1 in wild-type and Zmpste24 −/− MEFs and in kidney from wild-type and Zmpste24 −/− mice. ( d ) Quantification of experiments in c . Data represent mean±s.e.m., n =3. * P< 0.05, two-tailed t -test. ( e ) Representative immunoblots showing levels of different histone modifications in total cell lysate from wild-type and Zmpste24 −/− MEFs and indicated wild-type and Zmpste24 −/− tissues. ( f ) Quantification of experiments in e . Data represent mean±s.e.m., n =3. * P< 0.05, two-tailed t -test. ( g ) Representative photos of immunofluorescence staining of H3K9me3 in wild-type and Zmpste24 −/− MEFs. Scale bar, 20 μm. Full size image Global level of trimethylated H3K9 is mainly catalysed by Suv39h1/2 methyltransferases, of which Suv39h1 is ubiquitously expressed, whereas Suv39h2 is mainly observed in testis [21] . To investigate whether H3K9me3 is affected in Zmpste24 –/– MEFs, level of H3K9me3 was examined and compared between Zmpste24 –/– MEFs and wild-type littermates. As shown in Fig. 2e , the level of H3K9me3 was significantly increased in Zmpste24 –/– MEFs and tissues (kidney and lung) compared with that in littermate wild-type controls. In addition, the level of H4K20me3 was also significantly elevated in Zmpste24 –/– MEFs compared with wild-type controls, whereas H3K27me3 and H3K9me2 were hardly affected ( Fig. 2e ). The elevated H3K9me3 in Zmpste24 –/– MEFs was further confirmed by immunofluorescence microscopy ( Fig. 2g ). The increase in levels of H3K9me3 and H4K20me3 in Zmpste24 –/– MEFs was most likely attributable to unprocessed prelamin A, as ectopic unprocessible prelamin A (hereafter, prelamin A) led to similar upregulation in HEK293 cells ( Fig. 3 ). Therefore, the accumulation of prelamin A and progerin results in increased H3K9me3. 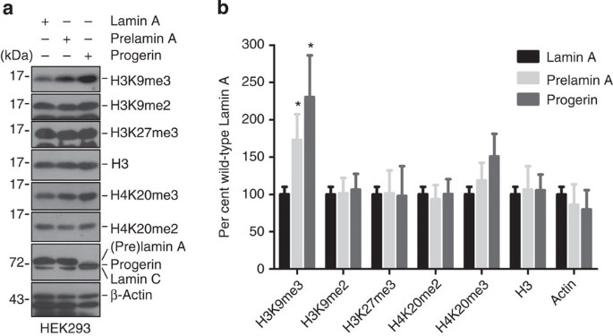Figure 3: Heterochromatic histone modifications in HEK293 cells with different ectopic lamins. (a) Representative western blotting in total cell lysate from HEK293 cells expressing ectopic lamin A, prelamin A or progerin. (b) Quantification of experiments ina. Data represent mean±s.e.m.,n=3. *P<0.05, two-tailedt-test. Figure 3: Heterochromatic histone modifications in HEK293 cells with different ectopic lamins. ( a ) Representative western blotting in total cell lysate from HEK293 cells expressing ectopic lamin A, prelamin A or progerin. ( b ) Quantification of experiments in a . Data represent mean±s.e.m., n =3. * P< 0.05, two-tailed t -test. Full size image The increased level of H3K9me3 in Zmpste24 –/– MEFs and cells with ectopic progerin seems discordant to previous reports on HGPS fibroblasts mainly determined by immunofluorescence staining [22] , [23] , [24] . It has been shown that the reduced H3K9me3 is a late event [24] , suggesting that the downregulation of H3K9me3 in HGPS cells might be secondary due to extensive in vitro passaging. To test this possibility, we re-examined and compared the level of H3K9me3 in six lines of fibroblasts isolated from 2- to 8-year-old HGPS patients, fibroblasts isolated from a 7-month-old healthy boy (PH) and a 3-month-old foetus (F2-S), at passage 12. Compared with PH cells, three out of six HGPS fibroblast cell lines, that is, HGADFN155, HGADFN164 and HGADFN188, showed upregulation of H3K9me3, while HGADFN143 and HGADFN169 showed obvious downregulation of H3K9me3; meanwhile, HGADFN122, HGADFN155, HGADFN164 and HGADFN188 showed an increase in H4K20me3 ( Fig. 4a ). The level of H3K9me3 seemed negatively associated with the donor age among healthy individuals or HGPS patients ( Fig. 4b ). This prompted us to further compare PH with an age- and gender-matched HGPS cell line HGADFN003 (HG003) derived from a 2-year-old male HGPS patient at different passages. As shown in Fig. 4c , H3K9me2, which normally marks transcriptionally silent euchromatic region [25] , didn’t exhibit significant alteration at different passages or between PH and HG003 cells within the passages examined. In contrast, levels of H3K9me3 and H4K20me3 decreased significantly with passage in both PH and HG003 cells. When compared with PH cells at the same passage, relatively higher levels of H3K9me3 and H4K20me3 were observed in HG003 cells ( Fig. 4c ). Similar to H3K9me3, an overall increase in H4K20me3 staining was observed in HG003 when compared with that in PH, whereas changes in the euchromatic H3K4me3 and H3K9ac were hardly observed ( Fig. 4e and Supplementary Fig. S4 ). H3K9me3 staining was found to be enriched in nuclear compartments ( Fig. 4e , arrows), wherein no typical DAPI staining of senescence-associated heterochromatin foci (SAHF, a hallmark of oncogene-induced senescence) were observed [26] , [27] , [28] . This is consistent with a recent report showing lack of SAHF in HGPS cells [29] . These data suggest opposing effects of prelamin A/progerin and passages on the regulation of H3K9me3 in primary human cells. Therefore, it is of particular importance to take passage into consideration in addition to age, sex and location of the skin sampling and so on, when determining heterochromatin marks in progeria. ‘Perfectly’ matched samples are essential for a reliable conclusion. To circumvent this problem, we examined levels of these heterochromatic marks in HEK293 cells expressing ectopic wild-type lamin A, prelamin A or progerin. As shown in Fig. 3a , while levels of H3K9me2 and H3K27me3 were hardly affected by different A-type lamins, levels of H3K9me3 and H4K20me3 were significantly elevated in the presence of progerin or prelamin A, compared with that expressing ectopic lamin A, suggesting that prelamin A and progerin cause elevated H3K9me3. 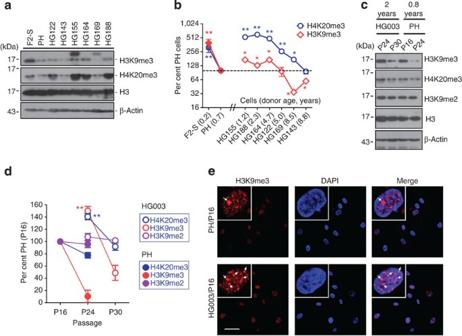Figure 4: Heterochromatic histone modifications in HGPS cells. (a) Representative western blotting showing levels of heterochromatic H3K9me3 and H4K20me3 in HGPS dermal fibroblast cell lines HGADFN122 (HG122), HGADFN143 (HG143), HGADFN155 (HG155), HGADFN164 (HG164), HGADFN169 (HG169) and HGADFN188 (HG188) derived from six individuals and aged from 2 to 8 years, PH and human fibroblasts from a 5-month foetus (F2-S). All cell lines were at passage 12. (b) Relative levels of histone modifications in various cells shown ina. Data represent mean±s.e.m.,n=3. *P<0.05, **P<0.01, two-tailedt-test, HGPS versus PH and F2-S versus PH. (c) Representative western blotting of H3K9me3 and H4K20me3 in human dermal fibroblasts HGADFN003 (HG003) derived from a 2-year-old male HGPS patient and PH cells from a healthy 7-month-old male at different passages. (d) Quantification of levels of histone modifications in experiments inc. Data represent mean±s.e.m.,n=3. **P<0.01, two-tailedt-test, HG003 (P24) versus PH (P24). (e) Immunofluorescence staining of H3K9me3 in PH and HG003 cells. Arrows show H3K9me3-enriched nuclear compartment. Scale bar, 40 μm. Figure 4: Heterochromatic histone modifications in HGPS cells. ( a ) Representative western blotting showing levels of heterochromatic H3K9me3 and H4K20me3 in HGPS dermal fibroblast cell lines HGADFN122 (HG122), HGADFN143 (HG143), HGADFN155 (HG155), HGADFN164 (HG164), HGADFN169 (HG169) and HGADFN188 (HG188) derived from six individuals and aged from 2 to 8 years, PH and human fibroblasts from a 5-month foetus (F2-S). All cell lines were at passage 12. ( b ) Relative levels of histone modifications in various cells shown in a . Data represent mean±s.e.m., n =3. * P< 0.05, ** P< 0.01, two-tailed t -test, HGPS versus PH and F2-S versus PH. ( c ) Representative western blotting of H3K9me3 and H4K20me3 in human dermal fibroblasts HGADFN003 (HG003) derived from a 2-year-old male HGPS patient and PH cells from a healthy 7-month-old male at different passages. ( d ) Quantification of levels of histone modifications in experiments in c . Data represent mean±s.e.m., n =3. ** P< 0.01, two-tailed t -test, HG003 (P24) versus PH (P24). ( e ) Immunofluorescence staining of H3K9me3 in PH and HG003 cells. Arrows show H3K9me3-enriched nuclear compartment. Scale bar, 40 μm. Full size image Lamin A mediates Suv39h1 stability To further understand the regulatory role for lamin A in Suv39h1 and H3K9me3, we examined whether loss of lamin A affects Suv39h1 stability and level of H3K9me3. As shown in Fig. 5a–c ), H3K9me3 was consistently and significantly decreased in 2 independent lines of Lmna null MEFs compared with that from wild-type littermate controls, while no significant changes in levels of H3K27me3, H4K20me3, H3K9me, H3K9me2, H3K4me3, acetylated H4 or acetylated H3 was observed. Immunofluorescence microscopy further confirmed the specific downregulation of H3K9me3 in Lmna –/– cells ( Fig. 5d and Supplementary Fig. S5a–e ). However, both mRNA and protein levels of Suv39h1 were found to be decreased in Lmna –/– cells ( Fig. 5e and Supplementary Fig. S5f ). To distinguish effects of lamin A in the transcriptional and post-translational regulation of Suv39h1, we knocked down LMNA by siRNA in HEK293 cells where ectopic GFP-SUV39H1 driven by a CMV promoter was expressed. The level of GFP-SUV39H1 was examined by western blotting. As shown in Fig. 5g , levels of GFP-SUV39H1 and H3K9me3 were both significantly reduced when lamin A/C level was downregulated, indicating that lamin A/C stabilizes GFP-SUV39H1 protein. This notion was further confirmed by the increased degradation of Suv39h1 in Lmna –/– cells when protein synthesis was inhibited by cycloheximide (CHX). As shown in Fig. 5e , >50% of Suv39h1 was degraded in Lmna –/– cells within 10 h upon CHX treatment compared with <25% in wild-type cells. Further investigation demonstrated that lamin A could stabilize Suv39h1 and thus prevent it from proteasomal degradation, as incubation with proteasome inhibitor MG-132 increased the level of Suv39h1 in Lmna –/– cells ( Supplementary Fig. S5h ). This is in line with a recent report showing proteasomal degradation of SUV39H1 (ref. 30 ). 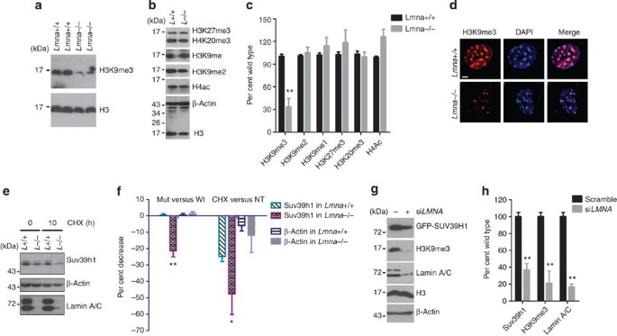Figure 5:Reduced levels of H3K9me3 and Suv39h1 inLmnanull cells. (a) Representative immunoblots in MEFs isolated from two pairs ofLmnanull and wild-type embryos, showing reduced level of H3K9me3. (b) Representative western blotting showing comparable levels of H3K27me3, H4K20me3, H3K9me1, H3K9me2 and acetyl H4 betweenLmnanull and wild-type cells. (c) Quantification of experiments inaandb. Data represent mean±s.e.m.,n=3. *P<0.05, two-tailedt-test. (d) Representative photos of immunofluorescence staining of H3K9me3 in wild-type andLmna–/–cells. Scale bar, 5 μm. (e) Representative immunoblots showing expression of Suv39h1 in wild-type andLmna–/–MEFs treated with CHX (10 μg ml−1). (f) Quantification of experiments ine. Left, per cent changes relative to wild-type cells; right, per cent changes relative to untreated (NT). Data represent mean±s.e.m.,n=3. *P<0.05, **P<0.01, two-tailedt-test. (g) Representative western blotting in HEK293 cells stably expressing GFP-SUV39H1 treated withLMNAor scramble siRNA. (h) Quantification of experiments ing. Data represent mean±s.e.m.,n=3. **P<0.01, two-tailedt-test. Figure 5: Reduced levels of H3K9me3 and Suv39h1 in Lmna null cells. ( a ) Representative immunoblots in MEFs isolated from two pairs of Lmna null and wild-type embryos, showing reduced level of H3K9me3. ( b ) Representative western blotting showing comparable levels of H3K27me3, H4K20me3, H3K9me1, H3K9me2 and acetyl H4 between Lmna null and wild-type cells. ( c ) Quantification of experiments in a and b . Data represent mean±s.e.m., n =3. * P< 0.05, two-tailed t -test. ( d ) Representative photos of immunofluorescence staining of H3K9me3 in wild-type and Lmna –/– cells. Scale bar, 5 μm. ( e ) Representative immunoblots showing expression of Suv39h1 in wild-type and Lmna –/– MEFs treated with CHX (10 μg ml −1 ). ( f ) Quantification of experiments in e . Left, per cent changes relative to wild-type cells; right, per cent changes relative to untreated (NT). Data represent mean±s.e.m., n =3. * P< 0.05, ** P< 0.01, two-tailed t -test. ( g ) Representative western blotting in HEK293 cells stably expressing GFP-SUV39H1 treated with LMNA or scramble siRNA. ( h ) Quantification of experiments in g . Data represent mean±s.e.m., n =3. ** P< 0.01, two-tailed t -test. Full size image Lamin A interacts with SUV39H1 Lamin A interacts with many nuclear proteins, that is, Rb, 53BP1 and ING1 and so on, thus preventing them from proteasomal degradation [31] , [32] , [33] . In addition, a recent elegant work by Bruston et al . [34] showed increased binding affinities of progerin and prelamin A, compared with lamin A, to histone H3 peptide trimethylated at K9. We reasoned that similar to H3K9me3, A-type lamins might directly or indirectly interact with SUV39H1, thus preventing it from degradation. Prelamin A/progerin may have increased binding capacity and protection on SUV39H1. To test this hypothesis, co-immunoprecipitation was performed in HEK293 cells expressing ectopic GFP-SUV39H1 and lamin A. Both GFP-SUV39H1 and lamin A were detected by western blotting in the anti-GFP immunoprecipitates ( Fig. 6a ). Endogenous SUV39H1 was observed in the anti-GFP immunoprecipitates in HEK293 cells where GFP-lamin A was ectopically expressed ( Fig. 6b ). The interaction between endogenous SUV39H1 and lamin A was confirmed in either anti-SUV39H1 or anti-lamin A/C immunoprecipitates in HEK293 cells, where SUV39H1 pulled down lamin A and vice versa ( Fig. 6c ). Confocal microscopy revealed the colocalization of GFP-SUV39H1 with DsRed-lamin A on the nuclear lamina as well as in the nucleoplasm ( Fig. 6d ), confirming the interaction between SUV39H1 and lamin A. Moreover, deletion of 89 amino acids (NΔ89) at the N-terminus of SUV39H1 completely abolished the interaction between GFP-lamin A and Myc-SUV39H1 in HEK293 cells ( Fig. 6e ). By co-immunoprecipitation with anti-lamin A antibodies in the test tube containing recombinant human lamin A (rhLamin A) and recombinant human SUV39H1 (rhSUV39H1), we found that rhLamin A co-precipitated with full-length rhSUV39H1 ( Fig. 6f ). Collectively, these results indicate that lamin A likely interacts with SUV39H1 via its N-terminal domains, possibly the chromo domain. 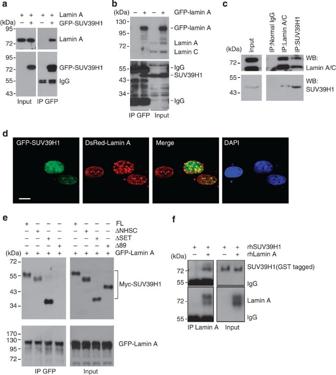Figure 6: Lamin A interacts with SUV39H1. (a) GFP-SUV39H1 and/or lamin A were ectopically expressed in HEK293 cells. Representative immunoblots showing ectopic lamin A in the anti-GFP immunoprecipitates. Data are representative of three independent experiments. (b) Representative immunoblots showing endogenous SUV39H1 in the anti-GFP immunoprecipitates in HEK293 cells expressing ectopic GFP-lamin A. (c) Representative western blotting of SUV39H1 and lamin A/C in the anti-SUV39H1 and anti-lamin A/C immunoprecipitates in HEK293 cells. (d) Representative photos of confocal microscopy in human fibroblasts expressing ectopic GFP-SUV39H1 and DsRed-lamin A, showing colocalization of DsRed-lamin A and GFP-SUV39H1 on the nuclear lamina and in the nuclear interior. Scale bar, 10 μm. (e) Representative western blotting showing various Myc-tagged SUV39H1 mutant proteins in the anti-GFP immunoprecipitates in HEK293 cells expressing GFP-lamin A and Myc-tagged SUV39H1 mutants. Note a complete loss of Δ89 in the anti-GFP immunoprecipitates. Abbreviations: FL, full-length SUV39H1; Δ89, N-terminal-89-amino-acid-deleted SUV39H1; ΔSET, SET-domain-deleted SUV39H1; ΔNHSC, NHSC-sequence-deleted SUV39H1. (f) Representative immunoblots showing full-length recombinant human SUV39H1 (rhSUV39H1) in the anti-lamin A immunoprecipitates in the test tube containing recombinant human lamin A (rhLamin A) and rhSUV39H1. Figure 6: Lamin A interacts with SUV39H1. ( a ) GFP-SUV39H1 and/or lamin A were ectopically expressed in HEK293 cells. Representative immunoblots showing ectopic lamin A in the anti-GFP immunoprecipitates. Data are representative of three independent experiments. ( b ) Representative immunoblots showing endogenous SUV39H1 in the anti-GFP immunoprecipitates in HEK293 cells expressing ectopic GFP-lamin A. ( c ) Representative western blotting of SUV39H1 and lamin A/C in the anti-SUV39H1 and anti-lamin A/C immunoprecipitates in HEK293 cells. ( d ) Representative photos of confocal microscopy in human fibroblasts expressing ectopic GFP-SUV39H1 and DsRed-lamin A, showing colocalization of DsRed-lamin A and GFP-SUV39H1 on the nuclear lamina and in the nuclear interior. Scale bar, 10 μm. ( e ) Representative western blotting showing various Myc-tagged SUV39H1 mutant proteins in the anti-GFP immunoprecipitates in HEK293 cells expressing GFP-lamin A and Myc-tagged SUV39H1 mutants. Note a complete loss of Δ89 in the anti-GFP immunoprecipitates. Abbreviations: FL, full-length SUV39H1; Δ89, N-terminal-89-amino-acid-deleted SUV39H1; ΔSET, SET-domain-deleted SUV39H1; ΔNHSC, NHSC-sequence-deleted SUV39H1. ( f ) Representative immunoblots showing full-length recombinant human SUV39H1 (rhSUV39H1) in the anti-lamin A immunoprecipitates in the test tube containing recombinant human lamin A (rhLamin A) and rhSUV39H1. Full size image Prelamin A and progerin stabilize SUV39H1 To test whether prelamin A and progerin have increased binding capacity to SUV39H1, we compared the interactions between GFP-SUV39H1 and different A-type lamins, that is, lamin A, prelamin A and progerin by co-immunoprecipitation. Interestingly, significantly more prelamin A and progerin were detected in the anti-GFP immunoprecipitates though comparable level of lamin A, prelamin A and progerin was found in the input and comparable GFP-SUV39H1 was pulled down ( Fig. 7a ), indicating increased binding capacity of SUV39H1 to prelamin A and progerin compared with lamin A. The different binding capacity among lamin A, prelamin A and progerin to SUV39H1 was further confirmed by a competitive co-immunoprecipitation where either prelamin A or progerin together with lamin A and GFP-SUV39H1 were co-transfected into HEK293 cells. The level of A-type lamins was determined in GFP-SUV39H1 pull-down by western blotting. The levels of lamin A and prelamin A/progerin were similar in the input. While pull-down RIPA buffer containing 500 mM NaCl completely abolished the interaction between A-type lamin and SUV39H1, GFP pull-down with RIPA containing 350 mM NaCl showed significantly more prelamin A or progerin than lamin A in the anti-GFP-SUV39H1 precipitates ( Fig. 7b ). 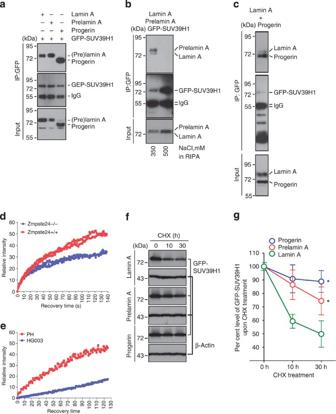Figure 7: Prelamin A/progerin stabilizes SUV39H1. (a) Representative immunoblots in the anti-GFP immunoprecipitates in HEK293 cells ectopically expressing GFP-SUV39H1 and one of the A-type lamins, that is, lamin A, prelamin A and progerin. Note that similar or lower level of prelamin A and progerin compared with lamin A were found in the input but significantly higher levels of prelamin A and progerin were pulled down, compared with lamin A. (b) Representative western blotting showing levels of lamin A and prelamin A pulled down by GFP-SUV39H1 in anti-GFP immunoprecipitates in HEK293 cells expressing ectopic GFP-SUV39H1, Lamin A and prelamin A. Note that the interaction between lamins and GFP-SUV39H1 was abolished at high concentration of NaCl (500 mM). The levels of prelamin A and lamin A were similar in the input. (c) Representative western blotting showing levels of lamin A and progerin pulled down by GFP-SUV39H1 in anti-GFP immunoprecipitates in HEK293 cells ectopically expressing GFP-SUV39H1, Lamin A and progerin. Note that the levels of progerin and lamin A are comparable in the input, whereas the level of progerin is significantly higher than that of lamin A in the GFP precipitates. (d,e) Representative FRAP data of GFP-SUV39H1 inZmpste24−/−versus wild-type MEFs (d) and PH versus HGADFN003 (HG003) cells (e). (f) Representative western blotting in CHX-treated GFP-SUV39H1 stably transfected HEK293 cells transiently expressing ectopic lamin A, prelamin A or progerin. (g) Quantification of experiments inf. Data represent mean±s.e.m. *P<0.05, two-tailedt-test, prelamin A versus lamin A and progerin versus lamin A. Figure 7: Prelamin A/progerin stabilizes SUV39H1. ( a ) Representative immunoblots in the anti-GFP immunoprecipitates in HEK293 cells ectopically expressing GFP-SUV39H1 and one of the A-type lamins, that is, lamin A, prelamin A and progerin. Note that similar or lower level of prelamin A and progerin compared with lamin A were found in the input but significantly higher levels of prelamin A and progerin were pulled down, compared with lamin A. ( b ) Representative western blotting showing levels of lamin A and prelamin A pulled down by GFP-SUV39H1 in anti-GFP immunoprecipitates in HEK293 cells expressing ectopic GFP-SUV39H1, Lamin A and prelamin A. Note that the interaction between lamins and GFP-SUV39H1 was abolished at high concentration of NaCl (500 mM). The levels of prelamin A and lamin A were similar in the input. ( c ) Representative western blotting showing levels of lamin A and progerin pulled down by GFP-SUV39H1 in anti-GFP immunoprecipitates in HEK293 cells ectopically expressing GFP-SUV39H1, Lamin A and progerin. Note that the levels of progerin and lamin A are comparable in the input, whereas the level of progerin is significantly higher than that of lamin A in the GFP precipitates. ( d , e ) Representative FRAP data of GFP-SUV39H1 in Zmpste24 −/− versus wild-type MEFs ( d ) and PH versus HGADFN003 (HG003) cells ( e ). ( f ) Representative western blotting in CHX-treated GFP-SUV39H1 stably transfected HEK293 cells transiently expressing ectopic lamin A, prelamin A or progerin. ( g ) Quantification of experiments in f . Data represent mean±s.e.m. * P< 0.05, two-tailed t -test, prelamin A versus lamin A and progerin versus lamin A. Full size image To further confirm the increased binding capacity between prelamin A/progerin and SUV39H1, we examined the mobility of SUV39H1, as increased association of SUV39H1 with prelamin A and progerin would decrease its mobility. Fluorescence recovery after photobleaching (FRAP) [35] was employed to compare the mobility of GFP-SUV39H1 between Zmpste24 −/− cells and wild-type controls. As shown in Fig. 7d , the recovery rate of GFP-SUV39H1 was significantly delayed in Zmpste24 −/− cells and HG003 cells compared with that in wild types or PH cells, suggesting that prelamin A and progerin have an enhanced association with SUV39H1 than lamin A, therefore the increased immobilization of SUV39H1. To test if the association of SUV39H1 with prelamin A/progerin protects it from degradation, lamin A or prelamin A or progerin were ectopically expressed in HEK293 cells stably expressing GFP-SUV39H1. Level of GFP-SUV39H1 was determined by western blotting after CHX treatment. While level of β-actin was quite stable in the presence of CHX for as long as 30 h, degradation of GFP-SUV39H1 is significantly faster in HEK293 cells transfected with lamin A compared with that with prelamin A or progerin ( Fig. 7f and Supplementary Fig. S6 ). The half-life of GFP-SUV39H1 in HEK293 cells transfected with empty vector, lamin A, prelamin A and progerin are ∼ 12 h, 23 h, 41 h and 48 h, respectively ( Supplementary Fig. S6 ). Collectively, these data implicated that prelamin A and progerin stabilize SUV39H1, leading to elevated SUV39H1 and H3K9me3 in progeroid cells. Depleting Suv39h1 ameliorates progeroid features in mice Given that either knocking down or depleting Suv39h1 rescued defective DNA repair, which is one of the potential underlying mechanisms of progeria, and critical roles for Suv39h1 and H3K9me3 in regulating heterochromatin repair and oncogene-induced senescence in mice [36] , we asked whether depleting Suv39h1 in Zmpste24 −/− mice could rescue accelerated cellular senescence, ameliorate progeroid features and extend lifespan. We crossed Zmpste24 −/− mice with Suv39h1 −/− mice to obtain Zmpste24 −/− Suv39h1 −/− compound mutant mice. Loss of Suv39h1 significantly rescued the shortened replicative lifespan in Zmpste24 −/− cells determined by a continuous passaging assay ( Fig. 8a ), and early senescence determined by senescence-associated β-galactosidase assay ( Fig. 8b ; 32.1%±9.8% β-galactosidase-positive cells in Zmpste24 −/− Suv39h1 −/− versus 65.7%±14.2% in Zmpste24 −/− MEFs, mean±s.e.m., P <0.05, two-tailed t -test). Similarly, knocking down Suv39h1/2 also rescued early senescence in Zmpste24 −/− MEFs ( Supplementary Fig. S7 ). 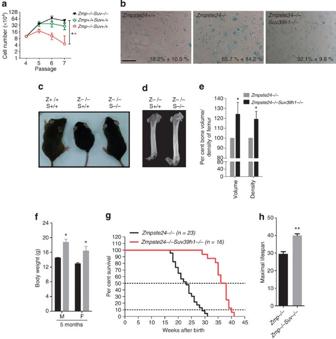Figure 8: Suv39h1 depletion ameliorates progeroid features and extends lifespan inZmpste24−/−mice. (a) Continuous passaging assay in MEFs showing extended replicative lifespan inZmpste24−/−Suv39h1−/−MEFs. Data represent mean±s.e.m.,n=3. **P<0.01, two-tailedt-test,Zmpste24−/−Suv39h1−/−versusZmpste24−/−MEFs. (b) Representative photos of β-galactosidase staining inZmpste24−/−Suv39h1−/−,Zmpste24−/−and wild-type MEFs. Percentages of β-galactosidase staining-positive cells were shown. Data represent mean±s.e.m.,n>200. Compound mutants exhibited significantly reduced percentages of β-galactosidase staining-positive cells (Zmpste24−/−Suv39h1−/−versusZmpste24−/−MEFs,P<0.05, two-tailedt-test). Scale bar, 200 μm. (c) Representative photo ofZmpste24+/+,Zmpste24−/−andZmpste24−/−Suv39h1−/−mice showing the partial rescue of body size at 4 months of age. (d) Representative microCT photos inZmpste24−/−andZmpste24−/−Suv39h1−/−mice at 4 months of age. (e) Bone volume and bone mineral density of femurs fromZmpste24−/−Suv39h1−/−mice andZmpste24−/−mice. Data represent mean±s.e.m.,n=3. *P<0.05, two-tailedt-test. (f) Body weight ofZmpste24−/−andZmpste24−/−Suv39h1−/−mice at 4 months of age. Data represent mean±s.e.m.,n=12. *P<0.05, two-tailedt-test. (g) Survival rate ofZmpste24−/−andZmpste24−/−Suv39h1−/−mice.P<0.0001. (h) Maximal lifespan (10% most long-lived animals) inZmpste24−/−andZmpste24−/−Suv39h1−/−mice. **P<0.01, two-tailedt-test. Figure 8: Suv39h1 depletion ameliorates progeroid features and extends lifespan in Zmpste24 − / − mice. ( a ) Continuous passaging assay in MEFs showing extended replicative lifespan in Zmpste24 − / − Suv39h1 − / − MEFs. Data represent mean±s.e.m., n =3. ** P< 0.01, two-tailed t -test, Zmpste24 − / − Suv39h1 − / − versus Zmpste24 − / − MEFs. ( b ) Representative photos of β-galactosidase staining in Zmpste24 − / − Suv39h1 − / − , Zmpste24 − / − and wild-type MEFs. Percentages of β-galactosidase staining-positive cells were shown. Data represent mean±s.e.m., n >200. Compound mutants exhibited significantly reduced percentages of β-galactosidase staining-positive cells ( Zmpste24 − / − Suv39h1 − / − versus Zmpste24 − / − MEFs, P< 0.05, two-tailed t -test). Scale bar, 200 μm. ( c ) Representative photo of Zmpste24 +/+ , Zmpste24 − / − and Zmpste24 − / − Suv39h1 − / − mice showing the partial rescue of body size at 4 months of age. ( d ) Representative microCT photos in Zmpste24 − / − and Zmpste24 − / − Suv39h1 − / − mice at 4 months of age. ( e ) Bone volume and bone mineral density of femurs from Zmpste24 − / − Suv39h1 − / − mice and Zmpste24 − / − mice. Data represent mean±s.e.m., n =3. * P< 0.05, two-tailed t -test. ( f ) Body weight of Zmpste24 − / − and Zmpste24 − / − Suv39h1 − / − mice at 4 months of age. Data represent mean±s.e.m., n =12. * P< 0.05, two-tailed t -test. ( g ) Survival rate of Zmpste24 − / − and Zmpste24 − / − Suv39h1 − / − mice. P <0.0001. ( h ) Maximal lifespan (10% most long-lived animals) in Zmpste24 − / − and Zmpste24 − / − Suv39h1 − / − mice. ** P< 0.01, two-tailed t -test. Full size image To examine whether loss of Suv39h1 ameliorates progeroid phenotypes, the body size, bone mineral density and lifespan were monitored accordingly. As shown, body size ( Fig. 8c ), bone volume, bone mineral density ( Fig. 8d ) and body weight ( Fig. 8f ) were significantly increased in Zmpste24 −/− Suv39h1 −/ mice compared with those in Zmpste24 −/− mice. Remarkably, the median survival was extended >60%, that is, from 23 weeks in Zmpste24 −/− mice to 37 weeks in Zmpste24 −/− Suv39h1 −/− mice ( Fig. 8g ). By 31 weeks after birth, all examined Zmpste24 −/− mice died, whereas more than 90% of Zmpste24 −/− Suv39h1 −/− mutants were still alive. The maximal lifespan (average lifespan of the most long-lived 10% of examined mice) was prolonged almost 40%, that is, 29 weeks in Zmpste24 −/− mice versus 40 weeks in Zmpste24 −/− Suv39h1 −/− mutants ( Fig. 8h ). Collectively, reducing H3K9me3 by depleting Suv39h1 significantly delayed the onset of premature aging in Zmpste24 −/− mice. These data suggest a regulatory role for heterochromatin regulation in senescence and premature aging. In the current study, we examined levels of Suv39h1 and H3K9me3 in HGPS dermal fibroblasts, Zmpste24 −/− cells and tissues and HEK293 cells expressing ectopic prelamin A and progerin. In comparison with lamin A, prelamin A and progerin exhibited elevated binding capacity to SUV39H1 thus increasing levels of SUV39H1 and H3K9me3 in progeroid cells. Depleting Suv39h1 specifically decreases the level of heterochromatic H3K9me3, leading to the rescue of defective DNA repair, early senescence and premature aging in Zmpste24 −/− mice. Our data for the first time demonstrated an interaction between lamin A and SUV39H1, suggesting a regulatory role for lamin A in the regulation of SUV39H1 methyltransferase and H3K9me3-mediated heterochromatin remodelling. As lamin A exists both on the nuclear periphery and in the nuclear interior, it is unclear which part(s) interact(s) with and stabilize(s) SUV39H1. On the other hand, lamin A directly interacts with many other proteins, such as lamin B1, to constitute the nuclear lamina and nuclear matrix, therefore the interaction between lamin A and SUV39H1 could be alternatively bridged by other proteins. Indeed, we found that SUV39H1 also directly or indirectly interacted with lamin B1 ( Supplementary Fig. S8 ). It is worth to mention that a direct interaction between recombinant lamin A and SUV39H1 was found in test tubes, suggesting the interaction between lamin A and SUV39H1 is most likely direct. Nevertheless, prelamin A/progerin exhibits increased binding capacity to SUV39H1; the C-terminus of prelamin A/progerin is likely responsible for the increased stability of SUV39H1 and level of H3K9me3 in progeria cells. Given that loss of Lmna in MEFs does not completely abolish H3K9me3, we reason that lamin A is not required for the initiation of H3K9me3. In addition to Suv39h1, lamin A directly interacts with H3 peptide containing trimethylated K9 (ref. 34) [34] ; therefore, it is plausible to speculate that initial H3K9me3 marks might facilitate recruiting chromatin to nuclear compartments wherein the lamin A-SUV39H1 complex resides and further trimethylates H3K9 on adjacent nucleosomes, thus expanding heterochromatic marks ( Supplementary Fig. S9 ). The increased H3K9me3 in progeria may seem discordant to previous reports [22] , [23] , [24] , while the rapid decline in levels of SUV39H1 and H3K9me3 along with passaging is in line with previous reports [24] , [37] . Our data showed that prelamin A/progerin and passage have opposing effects on the levels of Suv39h1 and H3K9me3 in progeroid cells. While prelamin A and progerin stabilize SUV39H1, thus increasing the level of H3K9me3 compared with lamin A, H3K9me3 decreases when passage goes up. This is in line with the finding that SUV39H1/2 transcript goes down with passage [24] . Therefore, caution must be taken when comparing HGPS cells with controls from healthy individuals, as in vitro passaging could significantly affect the results and the interpretation. In addition to H3K9me3, we found the level of H4K20me3, another constitutive heterochromatin mark, consistently upregulated in Zmpste24 −/− cells, HGPS dermal fibroblasts and HEK293 cells with ectopic prelamin A and progerin. It has been reported that Suv39h1 and H3K9me3 are required for the establishment of H4K20me3 and the recruitment of its methyltransferase Suv4-20H2 (refs 38 , 39 ). In this regard, the upregulation of H4K20me3 supports the increased H3K9me3 in progeroid cells. While accumulation of prelamin A in Zmpste24 null cells and ectopic prelamin A in HEK293 cells hardly affect the mRNA level of Suv39h1, loss of lamin A/C results in downregulation of Lmna transcription, suggesting a critical role for lamin A/C in regulating transcription. Meanwhile, it suggests that prelamin A likely preserve the transcriptional regulation of lamin A on SUV39H1, as only prelamin A exists in Zmpste24 −/− cells. Contrasting to Zmpste24 −/− mice, the SUV39H1 transcription has been shown downregulated in HGPS cells [24] . Given that ∼ 40% of lamin A is replaced with progerin in HGPS cells [40] , we speculate that while progerin exhibits similar function as prelamin A does in stabilizing SUV39H1 protein due to its abnormal carboxyl tail, it may loose parts of lamin A functions in the transcriptional regulation of SUV39H1, owing to the 50 amino-acid deletion. The level of SUV39H1 in HGPS fibroblasts might be a combined consequence of both transcriptional and post-translational regulations, for example, reduced transcription but increased protein stability. Therefore, the level of H3K9me3 in HGPS cells is a result of such regulations. To this point, our data are in line with previous report [24] . Supporting our findings and the gain-and-loss-of-function hypothesis is a recent study showing that prelamin A and progerin exhibited increased binding capacity to histone H3 peptide trimethylated at K9 in comparison with lamin A, while progerin reduced its binding capacity to DNA and H3 peptide containing either trimethylated or unmodified K27 compared with prelamin A and lamin A [34] . Deterioration of nuclear architecture is one of the hallmarks of laminopathy-based progeria. It has been shown that FTI treatment rescues the abnormal nuclear shape and thus alleviates progeroid features in progeria mouse models [8] , [11] , [12] . The rationale behind FTI treatment is largely based on the notion that the farnesylated carboxyl tail tethers prelamin A or progerin onto the nuclear lamina and thus jeopardizes the nuclear shape, and removal of the farnesyl group releases prelamin A or progerin from the nuclear lamina and thus rescues the nuclear shape and premature aging. However, a series of mouse lines with various mutation in Lmna have made things more complicated [41] . While farnesylation has been considered critical for nuclear envelop defects and progeroid phenotypes, mice with nonfarnesylated progerin may or may not elicit progeria [41] , [42] , [43] . On the other hand, expression of mature lamin A (18 amino acids deleted), bypassing the complicated prelamin A processing, deteriorates the nuclear shape but does not accelerate aging process in mice [44] . As different single-residue mutations could elicit quite different consequences, more stringent experimental design has been proposed to define the exact role of farnesylation in the development of progeria [43] . Nevertheless, our findings suggest an alternate mechanistic explanation that is independent of or parallel to envelope defect. It has been reported that defective DNA repair contributes, at least partially, to accelerated senescence in HGPS and progeroid mouse model [6] . In the current study, we have demonstrated that modulating heterochromatic H3K9me3 level by either deleting or knocking down Suv39h1 methyltransferase could rescue the defective DNA repair and delays the onset of premature aging in Zmpste24 −/− mice. Given that loss of Suv39h1 in mice does not result in any observable phenotype, modulating heterochromatin through Suv39h1 may provide an attractive additional approach for the intervention of HGPS. Collectively, our data suggest a direct or indirect interaction between lamin A and SUV39H1 and imply a role for lamin A in regulating one of the constitutive heterochromatic marks, H3K9me3. Our data also implicate a role for SUV39H1-mediated heterochromatin in laminopathy-based progeria and provide a potential therapeutic target for HGPS. Cell lines HEK293 cells, MEFs and human fibroblasts were maintained in DMEM supplemented with 10% FBS. HGADFN003 (HG003), HGADFN122 (HG122), HGADFN143 (HG143), HGADFN155 (HG155), HGADFN164 (HG164), HGADFN169 (HG169) and HGADFN188 (HG188) human dermal fibroblasts derived from HGPS patients were provided by Progeria Research Foundation (PRF). The PRF Cell and Tissue Bank is ‘Institutional Review Board approved by the Rhode Island Hospital Committee on the Protection of Human Subjects, Federal Wide Assurance FWA00001230, study CMTT#0146-09’ (cited from PRF official website: http://www.progeriaresearch.org/cell_tissue_bank.html ). Human PH dermal fibroblasts were from Professor Manfred Wehnert (Institute of Human Genetics, University of Greifswald, Greifswald, Germany). F2-S human fibroblasts were described previously [6] . Plasmids and siRNA transfections Plasmid and siRNA transfection was performed with Lipofectamine2000 (Invitrogen, USA) according to the manufacturer’s procedures. Sequences of siRNA oligonucleotides are as follows, SUV39 siRNA, 5′-ACCUCUUUGACCUGGACUA-3′; LMNA siRNA, 5′-CUGGACUUCCAGAAGAACA-3′. Lamin A, unprocessible prelamin A and progerin constructs were generated by bacterial recombineering. GFP-SUV39H1 construct is a gift from Dr CM Wong (Department of Pathology, The University of Hong Kong). Constructs of full-length and mutated Myc-SUV39H1 were provided by Dr Danny Reinberg (Howard Hughes Medical Institute; NYU School of Medicine Smilow Research Center, New York, USA). Antibodies Rabbit anti-Suv39h1 (1:500 dilution) and histone H3 (1:10,000 dilution) antibodies were obtained from Abcam (Cambridge, UK). Anti-lamin A/C (1:3,000 dilution for western blotting; 1:100 dilution for immunofluorescence staining) and 53BP1 (1:50 dilution for immunofluorescence staining) antibodies were purchased from Santa Cruz Biotechnology (Santa Cruz, CA, USA). Mouse anti-Suv39h1 (1:500 dilution), rabbit anti H3K9me3 (1:1,000 dilution for western blotting; 1:50 dilution for immunofluorescence staining), H3K9me2 (1:1,000 dilution), H3K27me3 (1:1,000 dilution), H4K20me3 (1:3,000 dilution), H4K20me2 (1:1,000 dilution), H3K9ac (1:1,000 dilution) and acetyl H3 (1:1,000 dilution) antibodies were sourced from Millipore (Bedford, MA, USA). Mouse anti-GFP (1:3,000 dilution) antibodies were purchased from Roche (Indianapolis, IN, USA). SA-β-galactosidase assay in MEFs was performed using a Cellular Senescence Assay Kit (Chemicon International, CA, USA), according to the manufacturer’s instructions. Unless otherwise mentioned, dilution factors are indicated for western blotting. Zmpste24 −/− Suv39h1 −/− mice Zmpste24 –/– mice have been described previously [5] . Suv39h1 −/− mice were provided by Dr Thomas Jenuwein (then at the Research Institute of Molecular Pathology, IMP, in Vienna). Zmpste24 –/– mice were crossed to Suv39h1 –/– mice to get Zmpste24 –/– Suv39h1 –/– mice. Body weight and lifespan of Zmpste24 −/− and Zmpste24 −/− Suv39h1 −/− mice was recorded. Bone mineral density was determined by MicroCT. The survival rate was analysed by Kaplan–Meier method and statistical comparison was performed by Log-rank (Mantel-Cox) Test. Mouse experimentation was performed in accordance with the guidelines of the Committee on the Use of Live Animals in Teaching and Research (CULATR) at the University of Hong Kong. Western blotting and Co-immunoprecipitation Whole-cell lysate was prepared by suspending the cells in 1 volume of suspension buffer (10 mM Tris-HCl, pH 7.5, 0.1 M NaCl, 1 mM EDTA, 1 mM DTT, pH 8.0, protease inhibitors), and then adding 1 volume of Laemmli buffer (0.1 M Tris-HCl, pH 7.0, 4% SDS, 20% glycerol, 1 mM DTT, protease inhibitors) and boiling for 5 min. Western blotting was performed as described previously [6] . Relative band intensity was measured by Image J and normalized to corresponding controls as indicated. For statistical analysis, at least three independent immunoblots were quantified and two-tailed t -test was used for P -values. For co-immunoprecipitation, cells were lysed into pre-chilled RIPA buffer with 300 mM NaCl. Primary antibody or appropriate control IgGs was added to the lysate and incubated for 2 h on a rocking platform at 4 °C before agarose beads were added and incubated overnight. The beads were washed twice with RIPA buffer, resuspended into Laemmli buffer and boiled and protein suspension was collected by centrifugation and stored for further analysis. For direct protein–protein interaction, co-immunoprecipitation was performed with 2–5 μg antibodies in the test tube containing recombinant human lamin A (Abcam, Cambridge, UK) and full-length recombinant human rhSUV39H1 (SignalChem, Richmond, Canada). Full-length images of immunoblots are shown in Supplementary Fig. S10 . Immunofluorescence staining Cells grown on chamber-slides were washed with PBS and fixed in 4% paraformaldehyde. Slides were blocked in 1% BSA/PBS with 5% normal host serum overnight at 4 °C, and then incubated with primary antibody diluted in 1% BSA/PBS overnight at 4 °C in a humid box. The slides were washed three times with PBS, incubated with FITC- or TRITC-coupled secondary antibodies diluted in 1% BSA/PBS for 40 min at room temperature., washed three times with PBS to remove unbound antibodies, mounted with SlowFade Gold antifade reagent with DAPI (Invitrogen, USA), sealed with nail polish and subjected for microscopy analysis. Photos were processed with Photoshop CS. Two-tailed t -test was used for P -values where applied. FRAP analysis FRAP was done as described [45] with a few modifications. Briefly, MEFs were plated on glass-bottom Petri dishes and GFP-SUV39H1 was transfected with lipofectamine2000 according to the manufacturer’s instructions. Forty-eight hours after transfection, FRAP was performed in a 37 o C/5% CO 2 chamber using the 488-nm laser on a confocal microscope (LSM 510). Targeted cells were scanned five times before a single bleach of a region of interest (ROI) at full laser power. Time-lapse images were collected at 1-s intervals for up to 2 min. The fluorescence intensity of ROI was normalized to reference ROI (same size as ROI and in the same nucleus except no bleaching was applied) and background (outside the cell). The relative ROI fluorescence intensities were plotted as a function of time. How to cite this article: Liu B. et al . Depleting the methyltransferase Suv39h1 improves DNA repair and extends lifespan in a progeria mouse model. Nat. Commun. 4:1868 doi: 10.1038/ncomms2885 (2013).